Evolutionary differentiation of androgen receptor is responsible for sexual characteristic development in a teleost fish Teleost fishes exhibit complex sexual characteristics in response to androgens, such as fin enlargement and courtship display. However, the molecular mechanisms underlying their evolutionary acquisition remain largely unknown. To address this question, we analyse medaka ( Oryzias latipes ) mutants deficient in teleost-specific androgen receptor ohnologs ( ara and arb ). We discovered that neither ar ohnolog was required for spermatogenesis, whilst they appear to be functionally redundant for the courtship display in males. However, both were required for reproductive success: ara for tooth enlargement and the reproductive behaviour eliciting female receptivity, arb for male-specific fin morphogenesis and sexual motivation. We further showed that differences between the two ar ohnologs in their transcription, cellular localisation of their encoded proteins, and their downstream genetic programmes could be responsible for the phenotypic diversity between the ara and arb mutants. These findings suggest that the ar ohnologs have diverged in two ways: first, through the loss of their roles in spermatogenesis and second, through gene duplication followed by functional differentiation that has likely resolved the pleiotropic roles derived from their ancestral gene. Thus, our results provide insights into how genome duplication impacts the massive diversification of sexual characteristics in the teleost lineage. Vertebrates exhibit a great variety of sexually dimorphic morphological and behavioural traits that are thought to have evolved through sexual selection. Sexual dimorphism in vertebrates has been extensively studied in rodents, especially in the context of male-biased sexual characteristics, such as external genitalia, sex accessory organ development, and reproductive behaviours [1] , [2] . However, few empirical studies have investigated the molecular mechanisms underlying the evolutionary acquisition of diverse sexually dimorphic traits in vertebrates. Teleosts show extreme sexual dimorphism [3] , such as an elongated median fin [4] , copulatory organs [5] , [6] , and nuptial coloration [7] , and behavioural traits including nest building [8] , courtship [9] , and aggressive acts [10] . Such male traits increase male reproductive success but often harm females because of the sex-specific fitness optima of these traits. Therefore, the genetic correlation between the two sexes constrains the evolution of sexual dimorphism, which generates intra-locus sexual conflict [11] , [12] . Although male-biased gene expression by androgens is a possible mechanism to resolve such sexual conflict by allowing the expression of morphological and behavioural traits specifically in mature male vertebrates [13] , [14] , [15] , [16] , little is known about the relationship between the genetic programme regulated by androgens and the evolutionary diversification of sexually dimorphic traits. Phenotypic and physiological responses to androgens are mediated by the androgen receptor (Ar), which belongs to the nuclear receptor family, a diverse group of transcription factors that originated in multicellular animals [17] , [18] , [19] , [20] . The Ar is composed of three major functional domains, a hypervariable N-terminal domain (NTD), a central highly conserved DNA binding domain (DBD) consisting of two zinc finger motifs, and a COOH-terminal ligand binding domain (LBD) [17] , [18] , [19] , [20] (Supplementary Fig. 1 ). In mammals, testosterone (T) and 5α-dihydrotestosterone are effective ligands for AR [21] . 11Ketotestosterone (11KT) is a potent androgen in teleosts [22] . Traditional studies using mouse models have shown that AR knockout ( AR KO) results in the demasculinisation of external genitalia, agenesis of accessory sex organs, and arrest of spermatogenesis [1] . Such pleiotropic functions [23] might have constrained the molecular evolution of the AR gene, although androgen-mediated gene expression can solve sexual conflict. Most teleosts have two distinct ar ohnologs —ara and arb— generated by teleost-specific whole-genome duplication (TSGD) [24] , [25] . The medaka ara and arb were mapped to chromosomes 10 and 14, respectively, with a conserved synteny relative to a single region locating the AR gene in human chromosome X, suggesting that the teleost ar gene duplication occurred as the result of TSGD [25] . TSGD is an evolutionarily recent whole-genome duplication that occurred ~350 Ma after the split of non-teleost actinopterygian lineages (namely, bichir, sturgeon, gar, and bowfin) from the teleost lineage, but before the divergence of Elopomorpha (i.e. Japanese eel) and Osteoglossomorpha (i.e. silver arowana) [26] , [27] . Because gene duplication results in a decrease in the negative selection pressure and can drive the establishment of lineage-specific traits with novel biological functions [28] , the ar ohnologs could have contributed to the diversification of masculine sexual characteristics found in teleosts, owing to the reduction of the pleiotropic constraint on them. Molecular evolutionary analysis of the teleost lineage has revealed the asymmetric evolution of ar ohnologs, including the accumulation of more novel substitutions in ara than in arb after the divergence of Elopomorpha, and that the lineage-specific loss of ara occurred independently in Otocephala such as zebrafish and Salmoniformes such as rainbow trout (Supplementary Fig. 1 ) [24] , [25] , [29] , [30] , [31] . Our in vitro analysis of the protein function of medaka Ars indicates that Arb has properties similar to those of other vertebrate Ars, but Ara acquired a new function as a hyperactive form of Ar, showing higher ligand-dependent transactivation capacity and constitutive nuclear localisation [25] . We also found two key nonsynonymous base substitutions in the Ar hinge region and LBD, which are highly conserved among spiny-rayed fish (Acanthomorpha) Aras, including medaka and cichlid Aras but not in Japanese eel Ara [30] . Such substitution in the hinge region has changed the molecular property of Ara from a ligand-dependent- to a constitutive-nuclear localisation protein, while the substitution in the LBD has increased its transactivation capacity [30] . This suggests that retention of the two Ar ohnologs with neofunctionalisation and/or subfunctionalisation in the Acanthomorpha lineage can significantly contribute to reproductive diversification. A recent genetic study in the African cichlid ( Astatotilapia burtoni ) revealed that the two Ar ohnologs have diverged in their functional roles for male sexual characteristics [32] . However, the molecular basis of how the two Ar ohnologs exhibit functional divergence has not yet been elucidated. To understand the molecular properties of Ar ohnologs in the diversification of sexual characteristics, we focused on the role of Ar in Japanese medaka ( Oryzias latipes ), which is a well-defined model system for the study of sex determination [33] and sexual differentiation studies on morphological and behavioural traits [10] , [34] , [35] , [36] , [37] , [38] . Medaka has a male heterogametic (XX/XY) system, in which dmy/dmrt1bY on the Y chromosome determines their sexes [33] . Importantly, they show prominent external morphologies specific to males, such as modification of the anal fin with papillary processes and formation of a fork in the dorsal fin [39] . These sexual characteristics can be induced by androgen administration [40] and are probably regulated by ligand-dependent transcriptional regulation of Ars [36] . Males perform courtship behaviours consisting of a sequence of stereotyped actions that are easily quantified [35] , [38] , [41] . The sequence begins with the male approaching and following the female closely. The male then performs a courtship display, in which he swims quickly in a circular pattern in front of the female. If the female accepts the male, the male grasps her with his fins (termed “wrapping”), and they quiver together until eggs and sperm are released (“spawning”). If the male is not accepted, she either rapidly moves away from the male or assumes a rejection posture [38] , [41] . Furthermore, previous studies demonstrated that Ars are expressed in the brain [42] and can control the sexually dimorphic expression of neuropeptides and biologically active nonapeptides [10] , [43] . Although these findings indicate that Ars are involved in a broad range of male-specific traits in medaka, the differential role of the two Ars remains unclear. This study aimed to understand how evolutionary differentiation of Ar ohnologs contributed to the development of sexual characteristics that increase male fitness in teleosts, which provides insights into the mechanisms of radiation of teleost fishes driven by sexual selection. In this work, we isolated medaka ara and arb mutants that had lost their ligand-dependent transactivation capacity from a medaka TILLING (targeting-induced local lesions in genomes) library and then comprehensively characterised the phenotypes of sexual characteristics in the single ar mutants ( ara KO or arb KO) and double knockout mutants ( ar DKO). We find that both ara and arb are required in males to achieve efficient reproductive success; ara and arb are functionally redundant in the regulation of courtship display but have divergent roles in other morphological and behavioural sexual characteristics. Unexpectedly, both ar ohnologs are not essential for spermatogenesis in medaka, which contrasts with the case of mouse Ar and may have permitted the ar evolution in teleosts by reducing part of the functional constraints on the gene(s). We also demonstrate that differences in transcriptional regulation and intracellular localisation could account for the divergent roles of ar ohnologs in the development of the sexual characteristics of teleosts. Screening of ara and arb knockout mutants (KOs) By screening the medaka TILLING library, we identified founders possessing nonsense mutations in exon 6 of ara (S507X) and exon 4 of arb (L503X) (Supplementary Fig. 2a–c ). These nonsense mutations lead to expression of the truncated protein products lacking the LBD that contains a key amino acid-substitution responsible for distinct transactivation responses of Ara and Arb in vitro [30] (Supplementary Fig. 2 ). These mutant alleles failed to mediate 11KT-induced transcription of androgen response element (ARE) reporter genes in COS7 cells, indicating that these mutations in ara and arb resulted in the loss of ligand-induced transactivation capacity (Statistical differences were assessed using two-sided Mann-Whitney U test (R version 4.2.0). * P < 0.05 (WT vs Ara mutant: W = 16, P = 0.02857; WT vs Arb mutant: W = 16, P = 0.02857, Supplementary Fig. 2d ). Therefore, we established ara -/- ( ara KO) and arb -/- ( arb KO) medaka strains carrying homozygous null mutations of ara and arb , respectively, by crossing these founders. Furthermore, a double homozygous mutant strain ( ara -/- ; arb -/- , i.e. ar DKO) was established by crossing ara KO and arb KO strains. Roles of the two Ars in testicular development and spermatogenesis To evaluate the influence of the Ar mutations on sex determination, we analysed the genetic sex by the amplification of dmy and then confirmed the gonadal sex by dissecting their gonads. All wild-type (WT) and mutant fish with a Y chromosome (XY chromosomes) had testes ( n = 10 in each genotype), indicating that Ar mutations did not cause sex reversal. To examine the role of Ar mutations in male fecundity, we bred ar KO males with WT females. Although both ara KO males and arb KO males were fertile, their frequencies of successful reproduction and average rates of fertilisation were significantly decreased (Fig. 1a, b ). No ar DKO males successfully bred with females under natural mating (Fig. 1a ). In contrast, all mutant females were fertile and displayed fertilisation rates similar to those of WT females (Supplementary Fig. 3 ). We hypothesised that the lack of successful mating in ar DKO males was caused by defects in testicular differentiation and spermatogenesis, as demonstrated in previous studies in AR KO mice [1] . However, we discovered that the Ar mutants showed no difference in testicular morphology, except the ara KO males exhibiting hypertrophic testes filled with mature sperm, which correlated with their higher gonad/body weight ratio (gonadal-somatic index; GSI) (Fig. 1c, d ). We found that even in ar DKO males, the testes contained mature sperms with tails in the seminiferous tubules (Fig. 1e ). Fig. 1: Deficiency of either ara or arb reduces the frequency of spawning but maintains normal spermatogenesis. a Frequency of mating tests in which a WT female laid eggs within 30 min after initiation of the mating. We used WT ( n = 11, total 60 matings) and ara KO males ( n = 14, total 76 matings) of the same litter, and WT ( n = 6, total 42 matings) and arb KO ( n = 6, total 41 matings) of the same litter, and ar DKO males ( n = 10, total 43 matings), as mating partners for the WT females. Details of mating tests utilised for this and following behavioural analyses were shown in Supplementary Table 2. 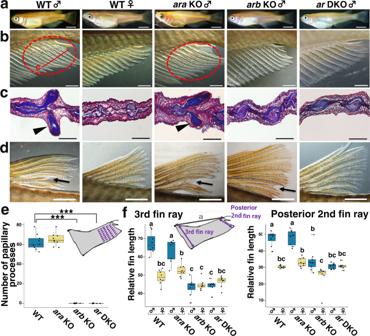Fig. 2:arbKO males andarDKO males display demasculinised fin structure, whereasaraKO males exhibit normal sexual characteristics in fin morphogenesis. aRepresentative picture of the whole body of WT male, WT female,araKO male,arbKO male, andarDKO males (n≥ 6 of each genotype). Higher magnification of the anal fin (b), the micrographs of Masson/trichrome-stained sections of anal fin (c), higher magnification of the dorsal fin (d) of WT males, WT females,araKO males,arbKO males, andarDKO males, respectively (n≥ 6 of each genotype). The papillary processes developments were marked by red dotted circles inband arrowheads inc. The plane of tissue section of anal fin is indicated by red line inb. Arrows indindicate forks in the dorsal fin.eNumber of developing papillary processes in adult WT,araKO,arbKO, andarDKO males (n= 9 for each genotype). The blue and light brown colours indicate WT andaraKO, respectively. The one-way ANOVA followed by two-sided Dunnett’s multiple comparison test indicates that the number of papillary processes was not decreased inaraKO (estimate ± s.e. = 2.667 ± 2.458,t= 1.085,P= 0.572) but completely absent inarbKO (estimate ± s.e. = −62.333 ± 2.458,t= −25.36,P< 1e-04) andarDKO (estimate ± s.e. = −62.333 ± 2.458,t= −25.36,P< 1e-04). ***P< 0.001.fLengths of the anterior 3rd and posterior 2ndanal fin rays relative to the anterior–posterior width (indicated as “a” in the picture) of the anal fin in WT,araKO,arbKO, andarDKO males and females (n= 8 for males and females of each genotype). The blue and light brown colours indicate males and females, respectively. Statistical differences were assessed using the two-way ANOVA followed by the Tukey–Kramer test. Different letters above the boxes indicate significantly different groups (P< 0.05, see Supplementary Table3for the statistical results). Scale bars ina,b,c, anddindicate 5.0 mm, 1.0 mm, 50 μm, and 1.0 mm, respectively. In the box-plots, the centre line indicates the median, box limits indicate the upper and lower quartiles, the whiskers indicate 1.5× interquartile range, and the points are outliers. Source data and statistical data are provided as aSource Datafile and Supplementary Table3, respectively. Means are shown. Different letters above the boxes indicate significantly different groups ( P < 0.05, two-sided Fisher’s exact test with Bonferroni correction: see Supplementary Table 3 for the statistical data.). 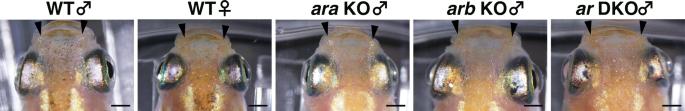Fig. 3:arbKO males andar DKOmales exhibited a diminished number of leucophores from nasal sacs to the dorsal side of the eyes, whereasaraKO males exhibit normal leucophore differentiation. Representative images of the upper jaw to the head of WT males, WT females,araKO males,arbKO males, andarDKO males (n= 5 for each genotype). Arrowheads indicate nasal sacs. Scale bars indicate 1 mm. b Percentage of fertilisation of ovulated oocytes from WT females in natural mating with WT, ara KO, and arb KO males ( n = 9, 7, and 6, respectively). The P values of fertilisation rates for natural mating ( b ) and artificial insemination ( i ) are calculated using two-sided Dunnett’s multiple comparison in a binomial GLMM (*** P < 0.001). c Gonad/body weight ratios of adult WT, ara KO, arb KO, and ar DKO males ( n = 6, 5, 5, and 4, respectively). The P values are calculated using two-sided Dunnett’s multiple comparison test. d Representative micrographs of Masson/trichrome-stained sections of adult gonads of WT males, WT females, ara KO males, arb KO males, and ar DKO males ( n ≥ 3 for each genotype). Scale bars represent 200 μm. e Higher magnification of Masson/trichrome-stained sections of WT testis and ar DKO testis. Scale bars represent 5 μm. f Number of sperm per testis of adult WT, ara KO, arb KO, and ar DKO males ( n = 6, 5, 5, and 4, respectively). The P values are calculated using two-sided Dunnett’s multiple comparison test ( f – h ), ** P < 0.01). g Percentage of sperm moving from WT, ara KO, arb KO, and ar DKO males ( n = 6, 5, 5, and 4, respectively). h Average speeds of sperm movement from WT, ara KO, arb KO, and ar DKO males ( n = 6, 5, 5, and 4, respectively). i Percentage of in vitro fertilisation of eggs from WT females using cryo-preserved sperm of WT, ara KO, arb KO, and ar DKO males ( n = 4 for each genotype). j Line drawing of a lateral view (anterior to the left) of the medaka urogenital region. The blue colour indicates the region of urogenital papillae (UGP) that prominently develops in the female. The red dotted line shows the approximate levels of the sections in k . k Representative micrographs of Masson/trichrome-stained sections of the urogenital region of WT males, WT females, ara KO males, arb KO males, and ar DKO males ( n ≥ 3 for each genotype). Scale bars represent 200 μm. The urethra, sperm duct, and enlarged medulla surrounding the sperm duct are indicated by *, red arrowhead, and red arrow, respectively. In the box-plots, the centre line indicates the median, box limits indicate the upper and lower quartiles, the whiskers indicate 1.5× interquartile range, and the points are outliers. The blue, light brown, dark brown, and grey colours indicate WT, ara KO, arb KO, and ar DKO, respectively. Source data and statistical data are provided as a Source Data file and Supplementary Table 3 , respectively. Full size image Sperm quality was examined using a computer-assisted sperm analysis system (CASA). Total sperm number was significantly increased in ar DKO males (two-sided Dunnett’s multiple comparison test: estimate ± s.e. = 5.4161 ± 1.5049, t = 3.599, P = 0.0067) and tended to increase in ara KO males (estimate ± s.e. = 1.7474 ± 1.4118, t = 1.238, P = 0.4944 (Fig. 1f ), while there were no significant differences in the frequency of moving sperm and average speed of sperm in all mutant strains (Fig. 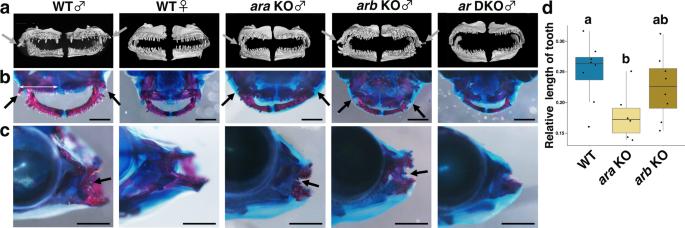Fig. 4:ar DKOmales have female-like teeth andaraKO males have a shorter lateral most tooth in the upper jaw, whereasarbKO males exhibit normal sexual characteristics in tooth morphogenesis. aMicro-CT images of the teeth (frontal view).b, cRepresentative images of bone staining of the teeth (n= 9 for each genotype). Arrow indicates the most lateral tooth. Scale bars indicate 1 mm.dLengths of the most lateral tooth relative to the lateral to medial width of the upper jaw stained with eosin (indicated as a line inb) in WT,araKO, andarbKO males (n= 8, 6, and 8, respectively). Statistical differences were assessed using one-way ANOVA, followed by two-sided Tukey’s multiple comparison test. Theargenotype significantly influenced the length of the tooth (one-way ANOVA, Df= 2,F= 3.796,P= 0.041). Two-sided Tukey’s multiple comparison test indicates that the length of the tooth was significantly decreased in thearaKO males (estimate ± s.e. = −0.07172 ± 0.02614,t= −2.744,P= 0.0327). Different letters above the boxes indicate significantly different groups (P< 0.05). The blue, light brown, and dark brown colours indicate WT,araKO andarbKO, respectively. In the box-plots, the centre line indicates the median, box limits indicate the upper and lower quartiles, the whiskers indicate 1.5× interquartile range, and the points are outliers. Source data and the other statistical data are provided as a Source Data file and Supplementary Table3, respectively. 1g, h ). Furthermore, no significant difference in the success rates of in vitro fertilisation using the cryopreserved sperms was found in all mutant strains (Fig. 1i ), These results indicate that all the mutant strains produce functional sperms that were capable of fertilising the eggs. Quantification of testicular levels of 11KT and T by liquid chromatography-mass spectrometry (LC/MS) revealed the ar genotype significantly affected the 11KT level (one-way analysis of variance (ANOVA), Df = 3, F = 26.58, P = 0.000164) but not the T and E2 levels (one-way ANOVA, T: Df = 3, F = 1.352, P = 0.325; E2: Df = 3, F = 2.007, P = 0.192. 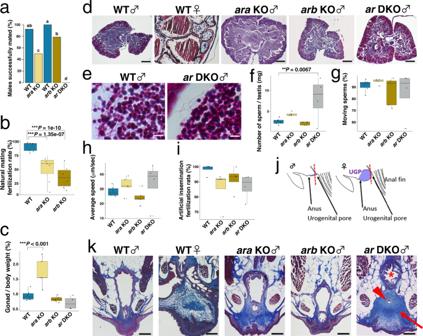The two-sided Dunnett’s multiple comparison test indicates that the 11KT level s was significantly increased in the ar DKO males (estimate ± s.e. = 65.417 ± 8.170, t = 8.007, P < 0.001) but not the ar single mutant males ( ara KO: estimate ± s.e. = 15.317 ± 8.170, t = 1.875, P = 0.218; arb KO: estimate ± s.e. Fig. 1: Deficiency of eitheraraorarbreduces the frequency of spawning but maintains normal spermatogenesis. aFrequency of mating tests in which a WT female laid eggs within 30 min after initiation of the mating. We used WT (n= 11, total 60 matings) andaraKO males (n= 14, total 76 matings) of the same litter, and WT (n= 6, total 42 matings) andarbKO (n= 6, total 41 matings) of the same litter, andarDKO males (n= 10, total 43 matings), as mating partners for the WT females. Details of mating tests utilised for this and following behavioural analyses were shown in Supplementary Table 2. Means are shown. Different letters above the boxes indicate significantly different groups (P< 0.05, two-sided Fisher’s exact test with Bonferroni correction: see Supplementary Table 3 for the statistical data.).bPercentage of fertilisation of ovulated oocytes from WT females in natural mating with WT,araKO, andarbKO males (n= 9, 7, and 6, respectively). ThePvalues of fertilisation rates for natural mating (b) and artificial insemination (i) are calculated using two-sided Dunnett’s multiple comparison in a binomial GLMM (***P< 0.001).cGonad/body weight ratios of adult WT,araKO,arbKO, andarDKO males (n= 6, 5, 5, and 4, respectively). ThePvalues are calculated using two-sided Dunnett’s multiple comparison test.dRepresentative micrographs of Masson/trichrome-stained sections of adult gonads of WT males, WT females,araKO males,arbKO males, andarDKO males (n≥ 3 for each genotype). Scale bars represent 200 μm.eHigher magnification of Masson/trichrome-stained sections of WT testis andarDKO testis. Scale bars represent 5 μm.fNumber of sperm per testis of adult WT,araKO,arbKO, andarDKO males (n= 6, 5, 5, and 4, respectively). ThePvalues are calculated using two-sided Dunnett’s multiple comparison test (f–h), **P< 0.01).gPercentage of sperm moving from WT,araKO,arbKO, andarDKO males (n= 6, 5, 5, and 4, respectively).hAverage speeds of sperm movement from WT,araKO,arbKO, andarDKO males (n= 6, 5, 5, and 4, respectively).iPercentage of in vitro fertilisation of eggs from WT females using cryo-preserved sperm of WT,araKO,arbKO, andarDKO males (n= 4 for each genotype).jLine drawing of a lateral view (anterior to the left) of the medaka urogenital region. The blue colour indicates the region of urogenital papillae (UGP) that prominently develops in the female. The red dotted line shows the approximate levels of the sections ink.kRepresentative micrographs of Masson/trichrome-stained sections of the urogenital region of WT males, WT females,araKO males,arbKO males, andarDKO males (n≥ 3 for each genotype). Scale bars represent 200 μm. The urethra, sperm duct, and enlarged medulla surrounding the sperm duct are indicated by *, red arrowhead, and red arrow, respectively. In the box-plots, the centre line indicates the median, box limits indicate the upper and lower quartiles, the whiskers indicate 1.5× interquartile range, and the points are outliers. The blue, light brown, dark brown, and grey colours indicate WT,araKO,arbKO, andarDKO, respectively. Source data and statistical data are provided as a Source Data file and Supplementary Table3, respectively. = 6.267 ± 8.170, t = 0.767, P = 0.788) (Table 1 ). Expression analysis of gonad-specific genes, vasa , P450c17 and gsdf , indicates that germ cells, Leydig cells, and Sertoli cells were formed in the testes of ar DKO as in ar single KOs (Supplementary Fig. 4 ). Table 1 LC/MS analysis of androgen and oestrogen in testes Full size table Next, to investigate whether there were any morphological defects in tissues involved in sperm release, we observed the tissue structure of the urethra, sperm duct, and medulla of urogenital papillae in histological sections of the cloaca of the Ar KO strains (Fig. 1j, k ). We found that the ara KO and ar DKO males showed a narrowed sperm duct cavity surrounded by medulla containing dense collagen fibres intensely stained by aniline blue, while the arb KO males showed a milder phenotype; the medulla developed in the posterior end of the sperm duct near the opening of the digestive tract (Supplementary Fig. 5 ). These results indicate that sperm duct constriction by the enlarged medulla may cause an increased number of sperm in the testes of ara KO and ar DKO males. The differential roles of the two Ars in the development of sexual characteristics The functional contributions of ara and arb to the development of external sexual characteristics were examined in ar KO strains (Fig. 2a–f ). The ara KO males showed prominent masculine sexual characteristics in median fin morphology, including the formation of papillary processes that develop as branched bone nodules derived from anal fin rays, elongated anal fin rays (Fig. 2b, c ), and forked dorsal fin with elongated rays (Fig. 2d ), as with the WT males. In contrast, arb KO and ar DKO males showed shorter anal fin rays without any papillary processes, as observed in WT females (Fig. 2b, c ). Quantitative assessment of the anal fin confirmed that papillary processes were lacking in the arb KO and ar DKO males but not in the ara KO males (Fig. 2e ). These results were consistent with changes in the expression level of lef1 , an androgen effector gene that is important for papillary process development [36] , which was significantly reduced in the anal fins of ar DKO males but not in those of ara KO males (two-sided Dunnett’s multiple comparison test, DKO: estimate ± s.e. = −14.915 ± 3.671, t = −4.062, P = 0.00931, ara KO: estimate ± s.e. = −4.013 ± 3.671, t = −1.093, P = 0.58592, arb: estimate ± s.e.= −9.84 ± 3.671, t = −2.68, P = 0.06707. Supplementary Fig. 6 ). We further quantified the outgrowth of anal fin rays by calculating the ratios of the length of the anterior 3rd and posterior 2nd fin rays to the width of the anal fin which was significantly larger in males than that in females of the WT (Fig. 2f ). Such sexual differences in the relative length of the fin rays were observed in the both fin rays of ara KO and the posterior 2nd fin rays of the arb KO (two-sided Tukey’s multiple comparison test, ara KO anterior 3rd: estimate ± s.e. = −10.9001 ± 2.1411, t = −5.091, P < 0.001, ara KO posterior 2nd: estimate ± s.e. = −14.8789 ± 2.1825, t = −6.817, P < 0.001; arb KO posterior 2nd: estimate ± s.e.= −9.2562 ± 2.1825, t = −4.241, P = 0.00202), but not in the anterior 3rd of the arb KO (1.2227 ± 2.1411, t = 0.571, P = 0.99909) and completely absent in both fin rays of the ar DKO males (anterior 3rd: estimate ± s.e.= 2.2646 ± 2.1411, t = 1.058, P = 0.96279, posterior 2nd: estimate ± s.e. = −0.1568 ± 2.1825, t = −0.072, P = 1 (Fig. 2f ). Similary, male-specific fork formation in the dorsal fin was observed in ara KO, in part, found in the arb KO but completely absent in the ar DKO males (Fig. 2d ). These results indicate that arb predominantly controls masculine characteristics in the median fins of medaka. Fig. 2: arb KO males and ar DKO males display demasculinised fin structure, whereas ara KO males exhibit normal sexual characteristics in fin morphogenesis. a Representative picture of the whole body of WT male, WT female, ara KO male, arb KO male, and ar DKO males ( n ≥ 6 of each genotype). Higher magnification of the anal fin ( b ), the micrographs of Masson/trichrome-stained sections of anal fin ( c ), higher magnification of the dorsal fin ( d ) of WT males, WT females, ara KO males, arb KO males, and ar DKO males, respectively ( n ≥ 6 of each genotype). The papillary processes developments were marked by red dotted circles in b and arrowheads in c . The plane of tissue section of anal fin is indicated by red line in b . Arrows in d indicate forks in the dorsal fin. e Number of developing papillary processes in adult WT, ara KO, arb KO, and ar DKO males ( n = 9 for each genotype). The blue and light brown colours indicate WT and ara KO, respectively. The one-way ANOVA followed by two-sided Dunnett’s multiple comparison test indicates that the number of papillary processes was not decreased in ara KO (estimate ± s.e. = 2.667 ± 2.458, t = 1.085, P = 0.572) but completely absent in arb KO (estimate ± s.e. = −62.333 ± 2.458, t = −25.36, P < 1e-04) and ar DKO (estimate ± s.e. = −62.333 ± 2.458, t = −25.36, P < 1e-04). *** P < 0.001. f Lengths of the anterior 3rd and posterior 2 nd anal fin rays relative to the anterior–posterior width (indicated as “a” in the picture) of the anal fin in WT, ara KO, arb KO, and ar DKO males and females ( n = 8 for males and females of each genotype). The blue and light brown colours indicate males and females, respectively. Statistical differences were assessed using the two-way ANOVA followed by the Tukey–Kramer test. Different letters above the boxes indicate significantly different groups ( P < 0.05, see Supplementary Table 3 for the statistical results). Scale bars in a , b , c , and d indicate 5.0 mm, 1.0 mm, 50 μm, and 1.0 mm, respectively. In the box-plots, the centre line indicates the median, box limits indicate the upper and lower quartiles, the whiskers indicate 1.5× interquartile range, and the points are outliers. Source data and statistical data are provided as a Source Data file and Supplementary Table 3 , respectively. Full size image We also examined another male sexual characteristic, the androgen-inducible increase in white pigment cells (leucophores) distributed from the nasal sac to the dorsal side of the eyes [44] . Gross observations showed that leucophores were decreased in the arb KO and ar DKO males but not in the ara KO males (Fig. 3 ), indicating that arb plays a critical role in the sexual differentiation of leucophore patterns. Fig. 3: arb KO males and ar DKO males exhibited a diminished number of leucophores from nasal sacs to the dorsal side of the eyes, whereas ara KO males exhibit normal leucophore differentiation. Representative images of the upper jaw to the head of WT males, WT females, ara KO males, arb KO males, and ar DKO males ( n = 5 for each genotype). Arrowheads indicate nasal sacs. Scale bars indicate 1 mm. Full size image Sexual dimorphism in tooth morphology such as larger lateral teeth of the upper and lower jaws in males [45] is another trait regulated by androgen in medaka [46] . We observed broken teeth in males, but not in females (Fig. 4a ), which might be damaged by male-male competition. In fact, when two males and one female were placed in the same tank, a male showed aggressive competition and attacked the lateral body of another male using its face (Supplementary Movie 1 ). Micron-scale computed tomography (micro-CT) and bone staining revealed that the ar DKO males did not show any enlarged lateral teeth, as in WT females (Fig. 4a–c ). Interestingly, while enlargement of the lateral teeth of the upper jaw was observed in the arb KO males as in WT males, less enlargement was detected in the ara KO males (indicated by arrows in Fig. 4a–c ). Quantitative measurement of the teeth length by calculating the ratio of the length of the largest tooth in the upper jaw to the width of the upper jaw revealed that the teeth length was significantly decreased in the ara KO males compared to the WT males (two-sided Tukey’s multiple comparison test, WT vs ara KO: estimate ± s.e. = −0.07172 ± 0.02614, t = −2.744, P = 0.0327), but not in the arb KO males (WT vs arb KO: estimate ± s.e. = −0.02544 ± 0.0242, t = −1.051, P = 0.5544) (Fig. 4d ). These results indicate that masculinisation of tooth morphology is predominantly regulated by ara . Fig. 4: ar DKO males have female-like teeth and ara KO males have a shorter lateral most tooth in the upper jaw, whereas arb KO males exhibit normal sexual characteristics in tooth morphogenesis. a Micro-CT images of the teeth (frontal view). b, c Representative images of bone staining of the teeth ( n = 9 for each genotype). Arrow indicates the most lateral tooth. Scale bars indicate 1 mm. d Lengths of the most lateral tooth relative to the lateral to medial width of the upper jaw stained with eosin (indicated as a line in b ) in WT, ara KO, and arb KO males ( n = 8, 6, and 8, respectively). Statistical differences were assessed using one-way ANOVA, followed by two-sided Tukey’s multiple comparison test. The ar genotype significantly influenced the length of the tooth (one-way ANOVA, Df= 2, F = 3.796, P = 0.041). Two-sided Tukey’s multiple comparison test indicates that the length of the tooth was significantly decreased in the ara KO males (estimate ± s.e. = −0.07172 ± 0.02614, t = −2.744, P = 0.0327). Different letters above the boxes indicate significantly different groups ( P < 0.05). The blue, light brown, and dark brown colours indicate WT, ara KO and arb KO, respectively. In the box-plots, the centre line indicates the median, box limits indicate the upper and lower quartiles, the whiskers indicate 1.5× interquartile range, and the points are outliers. Source data and the other statistical data are provided as a Source Data file and Supplementary Table 3 , respectively. Full size image Differential effects of the two Ars on mating behaviours Previous studies have shown that ar expression in the brain and the pituitary regulates the expression of several hormones that can control the reproduction and social behaviours in medaka [10] , [43] , [47] . Hence, we observed the mating behaviour of a test male (homozygotes for the WT, ara KO, arb KO, or ar DKO alleles) with a WT female (Supplementary Movies 2 – 6 , short movies showing representative cases for each genotype). The ar DKO males mostly abolished courtship displays during behavioural testing, whereas the single mutant males displayed courtships in over 90% of the tests (Fig. 5a ), indicating that either of the two ar s is sufficient for this mating behaviour. However, we found differential effects of the two ar s on the frequency of courtship displays before spawning, which is an index of male sexual motivation (Fig. 5b ). Although generalised linear mixed models (GLMM) showed no significant change in the frequency of courtship displays of the ara KO males (estimate ± s.e. = 0.1520 ± 0.1570, z = 0.968, P = 0.3419), the arb KO males showed significantly decreased frequency (estimate ± s.e. = −0.7641 ± 0.3297, z = −2.317, P = 0.03268) (Fig. 5b ). This difference indicates that the arb KO males have lower sexual motivation than the ara KO and WT males. Fig. 5: Both ara and arb are required for high male reproductive success. a Percentage of mating tests with different females in which a male exhibited courtship display within a 30 min test period. We used WT ( n = 11, total 59 matings) and ara KO males ( n = 14, total 76 matings) of the same litter, and WT ( n = 6, total 40 matings) and arb KO males ( n = 6, total 40 matings) of the same litter, and ar DKO males ( n = 10, total 43 matings) as mating partners for the WT females. The blue, light brown, dark brown, and grey colours indicate WT, ara KO, arb KO, and ar DKO, respectively. Means are shown. Different letters above the boxes indicate significantly different groups ( P < 0.05, two-sided f isher’s exact test with a Bonferroni correction). b Frequency of courtship displays before spawning. c Time required for spawning (mating latency). d Total number of wrapping rejections by female. e Duration of wrapping followed by spawning. For b to e , we used WT ( n = 11, total 55 mating) and ara KO males ( n = 13, total 38 matings) of the same litter and WT ( n = 6, total 42 matings) and arb KO males ( n = 6, total 32 matings) of the same litter. The blue and brown colours in panel b to e indicate WT and ar KO males, respectively. Statistical differences were assessed by likelihood ratio test with two-sided alternative hypothesis in GLMMs ( b – d ) and LMMs ( b – e ) * P < 0.05, ** P < 0.01, *** P < 0.001. In the box-plots, the centre line indicates the median, box limits indicate the upper and lower quartiles, the whiskers indicate 1.5× interquartile range, and the points are outliers. Source data and statistical data are provided as a Source Data file and Supplementary Table 3 , respectively. f RNA-seq of the whole brain with the pituitary in males. Venn diagram indicating overlap among inter-genotype differentially expressed genes (DEGs) (genes with >2-fold change in expression, false discovery rate (FDR) < 0.05). g–i Volcano plot with the log 2 fold-change on the x -axis and −log 10 of the p value on the y-axis in expression between WT and ar DKO males ( g ), WT and ara KO males ( h ), and WT and arb KO males ( i ). Each dot represents a single gene with differently expressed genes (DEGs)coloured (FDR < 0.05). The p values shown in the panels were calculated using two-sided Fisher’s exact test with no adjustments for the multiple comparisons. Full size image A previous study demonstrated that medaka females prefer males with longer median fins [48] ; therefore, we hypothesised that feminised fin morphology caused by arb deficiency but not by ara could affect female mate preferences. In contrast to our expectations, we found that both ara KO and arb KO males required significantly longer mating latency ( ara KO, GLMM, estimate ± s.e. = 0.5081 ± 0.2342, t = 2.17, P = 0.03163; arb KO, GLMM, estimate ± s.e. = 1.1429 ± 0.2645, t = 4.321, P = 0.001353) (Fig. 5c ). Consistently, the total number of wrapping rejections by the female was significantly increased in the case of both the ara KO (GLMM, estimate ± s.e. = 2.3981 ± 0.3685, z = 6.507, P = 4.32e-07) and arb KO males (GLMM, estimate ± s.e. = 1.6222 ± 0.4585, z = 3.538, P = 0.002858) (Fig. 5d ). These results indicate that deficiency of either of the two ar genes decreases mate preference by the females. Furthermore, to understand the behavioural roles of the papillary processes that are thought to enable males to rub and prevent females from escaping during wrapping for spawning [41] , we measured the duration of each wrapping event followed by egg spawning (Fig. 5e ). Linear mixed models (LMMs) showed that the duration time was significantly reduced in both the ara KO (estimate ± s.e. = −7.853 ± 2.147, t = −3.658, P = 0.001675) and arb KO males (estimate ± s.e. = −3.455 + 1.723, t = −2.005, P = 0.04403) (Fig. 5e ), indicating that not only fin morphology but also any defects caused by ara deficiency affected wrapping behaviour. Finally, to verify whether these behavioural defects caused by ar mutations decrease male reproductive success, we performed a mate choice test using two males—a WT male and an ar KO male—with a WT female. We found that both ara KO ( χ 2 = 23.458, df = 1, P = 1.277e-06) and arb KO males ( χ 2 = 12.224, df = 1, P = 0.0004718) successfully mated with females in significantly fewer trials compared to WT males (Supplementary Fig. 7 ), suggesting that both ara and arb are required for high reproductive fitness in males. Brain transcriptomic changes in ar KOs Because ar DKO males mostly abolished courtship displays, we performed RNA-seq analysis using whole brain tissues, including the pituitary, isolated from WT and ar DKO males to identify genes that regulate male courtship display. We identified 290 genes that were differentially expressed between the WT and ar DKO males. However, Gene Ontology (GO) enrichment analysis did not reveal significant enrichment of these genes in particular biological processes such as the regulation of social and reproductive behaviours (Supplementary Fig. 8 ). Identification of genes regulating the male courtship display would require identification of neurons that control the male reproductive behaviour and high-resolution gene expression analysis in such neurons. Next, we compared RNA-seq data from whole brain tissues of WT, ara KO, and arb KO males to identify genes responsible for behavioural changes in ar KOs. We identified 153 and 167 genes that were differentially expressed in ara KO and arb KO males, respectively, compared to WT males (Fig. 5f ). Although GO enrichment analysis did not reveal the significant enrichment of these genes in particular biological processes (Supplementary Figs. 9 and 10 ), 106 of 153 and 120 of 167 genes were identified to be differentially expressed between ara KO and arb KO males, respectively (Fig. 5f ). Among these genes, expression level of neuropeptide B a ( npba ), which is known to regulate the female reproductive behaviour [49] , was 5.17 and 3.98 times higher in the ar DKO and arb KO males compared to WT males, respectively (Fig. 5g, i ). Additionally, expression level of hsd17b12a , whose product catalyses the transformation of estrone (E1) into E2 [50] and 11-ketoandrostenedione (11KA4) to 11KT [51] , was significantly higher in the males of all ar KO strains compared to WT males (Fig. 5g–i ). We detected no up-regulation of ara in the arb KO and that of arb in the ara KO, which indicates that no detectable level of genetic compensation occurred between ara and arb at the whole-brain level. The quantification of steroid hormones by LC/MS revealed that the ar genotype significantly influenced the 11KT, T, E2, and E1 levels in the brains (one-way ANOVA, 11KT: Df = 3, F = 340.9, P = 8.90E-09; T: Df = 3, F = 24.42, P = 0.000222; E2: Df = 3, F = 4.724, P = 0.0352; E1: Df = 3, F = 6.351, P = 0.0164). The two-sided Dunnett’s multiple comparison test indicates that the 11KT and T levels were significantly increased in the ara KO and ar DKO males (11KT for ara KO, estimate ± s.e. = 1.373 ± 0.307, t = 4.474, P = 0.00524; 11KT for ar DKO, estimate ± s.e. = 8.38 ± 0.307, t = 27.3, P < 0.001; T for ara KO, estimate ± s.e. = 167.03 ± 48.89, t = 3.417, P = 0.0225; T for ar DKO, estimate ± s.e. = 320.33 ± 48.89, t = 6.553, P < 0.001) but not the arb KO males (11KT, estimate ± s.e. = 0.03 ± 0.307, t = 0.098, P = 0.99928; T, estimate ± s.e. = −57.2 ± 48.89, t = −1.17, P = 0.5393), whereas the E2 level was rather decreased in the arb KO and ar DKO males ( arb KO, estimate ± s.e. = −94.7 ± 32.59, t = −2.906, P = 0.0479; ar DKO, estimate ± s.e. = −95.57 ± 32.59, t = −2.963, P = 0.0442) (Table 2 ). These results indicate that arb predominantly represses the npba expression without inhibiting the E2 synthesis, whereas both ar ohnologs are required for repressing hsd17b12a expression in males, but ara is more effective in supressing 11KT and T synthesis. This is likely the reason why 11KT level increased in ara KO and ar DKO males. Such distinct roles for ar ohnologs in the regulation of Ar-biased gene expression in the brain may reflect the subfunctionalisation and/or neofunctionalisation of these ohnologs after the genome duplication event. Comparative genome sequence analysis combined with available ATAC-seq data in medaka [52] shows that putative cis -regulatory sequences of ara and arb , respectively, were partially conserved in teleost species, but not between ara and arb , supporting their subfunctionalization and/or neofunctionalization (Supplementary Fig. 11 ). Table 2 LC/MS analysis of androgen and oestrogen in brains Full size table Differences in expression and intracellular localisation of the two Ars To visualise expression patterns and intracellular localisation of Ara and Arb in vivo, we generated two knock-in medaka strains, ara FLAG-2A-mClover3 (Ara-KI) and arb FLAG-2A-mClover3 (Arb-KI) expressing two distinct proteins, an epitope (3xFLAG)-tagged Ar and a green fluorescent protein (mClover3), from the endogenous ar loci (Fig. 6a ). The Ara-KI adult males showed weak green fluorescence throughout the trunk and fins, and strong fluorescence in the regions adjacent to the pectoral, dorsal and anal fins. In contrast, the Arb-KI adult males showed a more restricted pattern of green fluorescence that localised primarily to the pectoral, dorsal and anal fins (Fig. 6b ). In the papillary processes of the anal fin, stronger green fluorescence was observed in Arb-KI than in Ara-KI males (Fig. 6b ). These differences in the expression patterns of Ara and Arb appear to be consistent with the results obtained from the comparative analysis of their cis -regulatory sequences (Supplementary Fig. 11 ). Next, we focused on the expression of Ara and Arb proteins in the cells located at the distal region of a bone nodule of papillary processes because we previously identified the expression of androgen effector genes in these cells [36] . We visualised Ara and Arb proteins in tissue sections of the anal fin by immunohistochemistry using a green fluorescent protein (GFP) antibody to identify the Ar-expressing cells and an anti-FLAG antibody to verify the nuclear localisation of Ar required for its activation as a transcription factor [53] . Consistent with the KO phenotype, we observed prominent GFP signals and nuclear localisation of FLAG signals in these Arb-KI cells, but not in Ara-KI cells (Fig. 6c ). These results suggest that the arb -specific gene expression and the nuclear localisation of arb protein in the papillary processes account for arb KO-specific defects in this tissue. Fig. 6: Visualisation of Ara and Arb expression in vivo by generating Ar-knock-in (KI) medaka strains. a Strategy for the generation of Ara and Arb KI medaka strains. We designed a gRNA targeting ara intron 8 and arb intron 7 (the last intron). In the donor plasmids, we cloned a genomic fragment beginning from the end of exon 8 of ara and exon 7 of arb and ending just before the stop codon in the last exon, exon 9 of ara , and exon 8 (shown as black closed boxes with ‘E8’) of arb , where the 3xFLAG sequences (shown as blue boxes) and a P2A (2A peptide from porcine teschovirus-1)-mClover3 cassette (shown as green boxes) was placed in the frame. Thus, endogenous Ara and Arb were expressed as FLAG fusion proteins. Both AR-FLAG and P2A-mClover3 were expected to be expressed under the control of the endogenous Ar promoter. To generate KI medaka, sgRNA (for genome digestion in the final intron), donor plasmid, and Cas9 mRNA were co-injected into one-cell-stage medaka embryos. After injection, concurrent cleavage of the targeted genomic locus and the donor plasmid resulted in the integration of donor plasmid DNA containing 3xFLAG-T2A-mClover3 by non-homologous end joining (NHEJ). The scheme shows the forward integration of 3xFLAG-T2A-mClover3. b Expression of mClover3 in adult males of the two knock-in medaka strains, ara FLAG-2A-mClover3 (Ara-KI) and arb FLAG-2A-mClover3 (Arb-KI). White, grey, and red arrows indicate the regions adjacent to pectoral, dorsal, and anal fins, respectively (Ara-KI). White, grey, and red arrows indicate the pectoral, dorsal, and anal fins, respectively (Arb-KI). c Immunohistochemical detection of FLAG-tagged endogenous Ara and Arb in longitudinal sections of papillary processes of the anal fin (6 μm thickness). The merged images represent red fluorescence for immunostaining of FLAG (anti-DDDDK-tag mouse mAb monoclonal antibody), green fluorescence for immunostaining of mClover3 (anti-GFP D5.1XP rabbit mAb monoclonal antibody), and blue fluorescence for nuclear staining by DAPI. The medaka Arb-FLAG, but not Ara-FLAG, translocated into the nuclei of cells located in the distal tip of a bone nodule of papillary processes (marked by white arrows). d Representative micrographs of Masson/trichrome staining and immunohistochemical detection of FLAG-tagged endogenous Ara and Arb in adjacent sections of the urogenital region (8 μm thickness). Nuclear localisation of Ara-FLAG and Arb-FLAG was observed in the medulla ventral to the sperm duct, where ar DKO exhibited hyperplasia. e, f Representative micrographs showing immunohistochemical detection of FLAG-tagged endogenous Ara and Arb, and DAPI counterstaining in the brain (12 μm thickness). f shows a higher magnification of the POA. Nuclear localisation of both Ara-FLAG and Arb-FLAG was observed in the POA. n = 6 for Ara-KI and Arb-KI males, respectively. Full size image In the urogenital region, nuclear localisation of both Ara and Arb was observed in the medulla ventral to the sperm duct (Fig. 6d ), where ar KOs exhibited prominent hyperplasia. In the preoptic area (POA), a brain region known to regulate a wide range of instinctive behaviours including mating behaviour [54] , we detected intense nuclear localisation of both Ara and Arb (Fig. 6e, f ). In the present study, we analysed the divergent roles of the TSGD-ohnolog pair ara and arb in the expression of sexual characteristics in medaka. We demonstrated that ar DKO males mostly abolished courtship displays and lacked external sexual characteristics, such as masculinisation of fin morphology and pigment cell patterns, resulting in infertility. These findings indicate the essential roles of Ars in male reproduction. Interestingly, ar DKO medaka showed successful spermatogenesis and no decrease in the number of mature sperms. This is consistent with the previous finding that medaka males deficient in the sex steroid synthesis-related gene P450c17 possess well-developed testes with many spermatozoa with fertilising ability [55] . Our results clearly showed that androgen signalling is dispensable for spermatogenesis in medaka. In contrast, impairment of spermatogenesis has been previously reported in Ar-deficient animals such as ARKO mice, in which spermatogenesis was arrested at the pachytene spermatocyte [1] and ar deficient zebrafish showing infertility due to defective spermatogenesis and/or release of sperm [56] , [57] , [58] . Additionally, the stimulatory effect of 11KT on spermatogenesis has been reported in cultured testes of Japanese eel, [22] which represents the earlier branching teleost groups [59] . These findings indicate that the functional contribution of androgen signalling to spermatogenesis has been lost, specifically in the lineage leading to medaka. Ar-mediated androgen activity also contributes to the maintenance of normal ovarian function in mouse [1] , [60] and zebrafish [56] , [57] , [58] . In contrast, Ar signalling is dispensable for female fecundity in medaka. The loss of contribution of Ar signalling in gametogenesis in both sexes might have reduced the evolutionary constraints on the ar ohnologs and accelerated the acquisition of exaggerated male-specific traits in the lineage leading to medaka. In fact, the medaka species that are widely distributed throughout southern and southeast Asia exhibit diversification of male-specific sexual characteristics in their fin morphology, pigmentation and behaviours [35] , [38] , [39] , [41] , [61] , [62] . To understand the exclusive role of ara and arb in the development of sexual characteristics, we analysed the morphological and behavioural traits of ara KO and arb KO males. We demonstrated that arb KO males showed a decreased frequency of courtship displays before spawning, reflecting their lower sexual motivation than WT males. In addition to such behavioural abnormalities, arb KO males lack external sexual characteristics, such as outgrowth of fin rays and papillary process development in the anal fin, as in females. Because females prefer males with longer fins [48] , and the papillary processes are thought to rub the female to induce spawning and prevent the females from escaping [41] , the demasculinisation of anal fin structure in arb KO males may reduce reproductive success. We also observed reduced reproductive success of the arb KO males due to the shorter duration of wrapping and subsequent spawning and rejection by females. This is consistent with the lower fertility caused by ablation of the part of the dorsal or anal fin in males [63] . In contrast, ara KO males showed intact sexual characteristics in fin morphogenesis but had shorter teeth. Although ara KO males did not show a decrease in sexual motivation considering the frequency of courtship displays before spawning, their frequency of mating was lower than that of WT males. Moreover, ara KO males were frequently subjected to wrapping rejection by females and exhibited a shorter duration of wrapping and subsequent spawning. These results indicate that their reproductive behaviour appears less attractive than that of WT males. In fact, ara KO males required more time to spawn with females. The lower fertility of ara KO males may be due to behavioural abnormalities as well as constriction of the sperm duct. Taken together, we revealed the differential roles of ar ohnologs associated with the sexual characteristics of teleosts— ara predominantly regulates the masculinisation of teeth and the reproductive behaviour eliciting female receptivity while arb plays essential roles in male-specific fin morphogenesis and sexual motivation. We confirmed that at least the phenotypes in fin morphogenesis and spermatogenesis in the ar TILLING KO medaka lines were reproduced by ar TALEN KO medaka lines (Supplementary Figs. 12 and 13 ), demonstrating that the observed phenotypes were not specific to the ar TILLING KO lines. Loss of function of either ara or arb reduced male reproductive fitness, whereas double mutations of ara and arb resulted in more severe phenotypes, indicating their overlapping and specific roles. The emergence of duplicated genes with overlapping roles that allow organisms to be phenotypically stable may relax selection pressure and enable innovation [64] , [65] , [66] , [67] . A recent study on African cichlid fish revealed that ara and arb diverged in their functions, wherein ara coded for reproductive and aggressive behaviours and arb for dominant bright colouration [32] . Corroborating this study, our findings suggest that external sexual characteristics, such as fin morphology and pigmentation patterns, are likely to be predominantly regulated by arb in both species. However, in contrast to the cichlid, the medaka ara regulates not only the performance of reproductive behaviour but also external sexual characteristics such as teeth enlargement that can be used in intra-male competition and the composition of medullary tissue in the cloaca, suggesting that the functional contribution of ara varies among species. A previous study comparing sequence differences between ara and arb showed that ara evolved 3.45 times faster than arb in medaka [30] . Taken together, these observations suggest that arb has been biased to maintain ancestral function under the stronger pressure of sexual selection compared to ara that has functionally diverged in each species. Further studies of other teleosts with two ar ohnologs and basal non-teleost ray-finned fishes (e.g. Polypterus) possessing a single ar gene are required to definitively determine the functions of ar ohnologs that have been derived from the ancestral gene and those that have been derived from innovated ar after the TSGD. So far, our previous analysis indicates that the Elopomorpha lineage including Japanese eel that represents the earlier branching teleost groups [59] , [68] have ar genes derived from ancestral genes before functional diversification, because the Japanese eel Ara and Arb did not show significant difference in their protein property in vitro [30] and have pleiotropic expression in various tissues such as testis, muscle, and spleen [69] . These observations suggest that the functional diversification of ar ohnologs has occurred in teleosts after the divergence of Elopomorpha lineage. The generation of epitope-tagged AR-KI medaka lines enabled us to analyse the accurate expression pattern of each Ar ohnolog in vivo. We found prominent expression of Arb, but not Ara, in the distal region of a bone nodule of papillary processes of the anal fin. In addition, we observed the localisation of Arb, but not Ara, in the cellular nuclei of this region. Such differential expression patterns of Ar ohnologs at the tissue and cellular levels may explain the loss of papillary processes in arb KO males. We also observed the cytoplasmic localisation of Ara in the anal fin, which appears to be inconsistent with a previous study showing constitutive nuclear localisation of Ara in COS-7 cells [25] . This may be explained by tissue- or cell type-specific expression of nuclear localisation signal (NLS)-binding proteins such as importin family proteins because Ara-specific amino acid substitution has been identified in its NLS that contacts the importin α proteins [30] . We observed the nuclear localisation of both Ara and Arb in other cells, such as the POA neurons of the brain and the medulla of the urogenital region. Together, these findings indicate that the differences in the regulation of both the transcription and intracellular localisation of Ars can become possible determinants of the functional differences of Ar ohnologs generated by TSGD. Identification of the downstream effector genes of Ars will enable us to reveal the genetic changes that underlie phenotypic novelty. Previous studies in mice have identified genes important for signalling pathways during developmental processes, including sonic hedgehog ( shh ), bone morphogenetic protein ( bmp ), and genes of the Wnt/β-catenin pathway [70] , [71] . Interestingly, we observed abnormal activation of neuropeptide B a ( npba ) and hsd17b12a expression, which were 5.17 and 4.12 times higher, respectively, in the brains of ar DKO males than in those of WT males (Fig. 5g ). npba is known as a downstream target of E2/Esr2b, which is necessary for female-specific mating behaviour [49] . Esr2b/E2 signalling plays a decisive role in the suppression of male-typical courtship display in females [38] . Besides, the expression of hsd17b12a has been shown to catalyse the transformation of E1 into E2 [50] . Therefore, we expected Esr2b signalling to be activated by increasing E2 levels in the brains of ar DKO males. However, contrary to our expectations, ar DKO males did not show any increase in brain E2 levels, indicating that the abnormal activation of npba expression in ar DKO males is not due to the rise in brain E2 levels and is maybe regulated by Ar signalling. Although we have not yet identified the downstream effector genes that account for each Ar-ohnolog-specific behaviour, we found that Ara and Arb have distinct repertoires of downstream effector genes in the brain. Abnormal activation of npba was exclusively found in arb KO males but not in ara KO males, suggesting that Arb has opposing effects on the expression of the female-biased gene necessary for female mating behaviour. Arb and Esr2b may interact competitively for the regulation of downstream effector genes. We aim to identify such genes in the future by conducting gene expression analysis in nerve nuclei with higher resolution and chromatin immunoprecipitation sequencing analysis of their target genes using the epitope-tagged AR-KI medaka lines generated in this study. In conclusion, we showed that in medaka, both ar ohnologs are not required for spermatogenesis but are required for high male reproductive success because of their overlapping and specific functions in the development of other male-specific morphological and behavioural sexual characteristics (Fig. 7 ). These findings suggest that the functional diversification of ar ohnologs has been promoted in the teleost lineage in two different ways—the loss of their roles in spermatogenesis and the gene duplication that has likely resolved the pleiotropic function derived from their ancestral gene. Furthermore, the generation of epitope-tagged AR-KI medaka lines enabled us to analyse the transcriptional regulation and intracellular localisation of each Ar, which filled a gap in knowledge, that is, the mechanism by which Ar ohnologs exhibit functional differences in vivo. Our results provide a comprehensive foundation for understanding the mechanisms underlying the diversification of sexual characteristics driven by ar gene duplication in teleosts. Fig. 7: Summary of the contribution of ara and arb to sexual characteristics. Based on the phenotypes of ara KO and arb KO, the contribution of each of the ar ohnologs to male sexual characteristics is indicated by + or −. For the characteristics regulated by both, the ar ohnolog that predominantly controls them is indicated by ++. Full size image Animals All the procedures and protocols were approved by the Institutional Animal Care and Use Committee of the National Institute for Basic Biology (15A005, 14A003, 13A023, 12A020, 11A028) and Kyushu University (A21-043-0, A19-137-0, A19-137-1, A19-137-2, A29-088-0, A29-088-1, A29-088-2). Japanese medaka ( Oryzias latipes ) were bred and maintained under artificial reproductive conditions with 14 and 10 h of light (8:00–22:00) and dark cycles at 26–28 °C. They were fed commercial pellet food (Hikari Lab; Kyorin Co., Ltd., Hyogo, Japan) 2–3 times a day. We used sexually matured (4–10 months old) male and female medaka producing fertilised eggs for at least three consecutive days until the day before the experiment. The ar DKO males were also reared with females in the same tank for one week until the day before the experiment. The gloss morphology and pigment pattern of the adult fish were observed using a stereo fluorescent microscope FLUO III TM (Leica, Wetzlar, Germany). Micrographs were taken using a digital charge-coupled device camera DP-73 (Olympus, Tokyo, Japan). Screening for ara and arb KOs from the medaka TILLING library In teleost fishes, two distinct subtypes of Ars were first identified as ARα and ARβ in Nile tilapia ( Oreochromis niloticus ), Japanese eel, and Atlantic croaker ( Micropogonias undulatus ) [69] , [72] , [73] . We have then distinguished the medaka Ars, ara (ARα, Genbank accession: AB252233, Ensembl ID: ENSORLG00000008220, located on chromosome 10), and arb (ARβ, AB252679, Ensembl ID: ENSORLG00000009520, located on chromosome 14), based on phylogenetic analysis considering those first identified as ARα and ARβ in Nile tilapia and Japanese eel [25] , [69] . Both ara KO and arb KO medaka strains were established using the TILLING approach. Briefly, the medaka TILLING library consisting of frozen sperm and genomic DNA obtained from 5760 F 1 male fish [74] was screened for mutations in ara and arb by high resolution melting (HRM) analysis [75] of fragments amplified by genomic PCR using KOD-Plus (Toyobo, Osaka, Japan) and ResoLight Dye (Roche, Mannheim, Germany) on a LightScanner System (96 software v2.0, Idaho Technology Inc., Salt Lake City, UT, USA). The PCR conditions for ara KO screening were as follows: preheating at 95 °C for 2 min, followed by 45 cycles of denaturation at 95 °C for 10 s, annealing at 58 °C for 30 s, and elongation at 68 °C for 30 s, and finally heating at 68 °C for 2 min. The conditions for arb KO screening were the same except the annealing temperature was set at 56 °C. The primer sequences used for KO screening are listed in Supplementary Table 1 . Fluorescence measurements were collected from 40 to 80 °C, and melting curves were analysed using the LightScanner System software version 2.0 (Idaho Technology Inc.). The PCR products selected as KO candidates were incubated with ExoSAP-IT reagent at 37 °C for 15 min, then inactivated at 80 °C for 15 min, and then directly sequenced on an ABI PRISM 3130xl Genetic Analyser (Life Technologies, Waltham, MA, USA) using a BigDye Terminator v3.1 cycle sequencing kit (Life Technologies). ID:5383 and ID:3793 were identified as founders harbouring nonsense mutations in the 6 th exon of ara ( ara S507X ) and the 4th exon of arb ( arb L503X ) (Supplementary Fig. 2 ). F 2 heterozygotes of KO males were obtained by artificial insemination using the National BioResource Project (NBRP) Medaka. To remove background mutations, heterozygous KO males were backcrossed with WT females of OK-Cab (NBRP ID: MT830) until the F 5 generation. After repeated backcrossing, the strains were maintained by crossing heterozygous females and males to obtain WT and homozygous siblings for phenotypic analyses. The ara and arb double heterozygous males and females ( ara +/− ; arb +/− ) were obtained by breeding ara −/− males with arb −/− females. The ara and arb double heterozygous males and females were crossed to obtain ara −/− ; arb +/− males and females. The ara and arb double homozygous males and females ( ara −/− ; arb −/− ) were obtained by breeding ara −/− ; arb +/− males with ara −/− ; arb +/− females. The genotype of each fish was determined by direct sequencing of the PCR product containing the mutant site from the fin clips of the adult fish using the same sets of primers for TILLING screening. The genetic sex of each fish was determined by genomic PCR according to a previous report [76] . Transcriptional activity of the Ar KO The expression vectors for medaka cDNAs for Ara (pCMV-medaka Ara + ) and Arb (pCMV-medaka Arb + ) were generated as previously described [30] , [77] . The mutations identified by TILLING were introduced into these expression vectors using the PrimeSTAR Max mutagenesis basal kit (Takara Bio, Shiga, Japan) and primers listed in Supplementary Table 1 to obtain pCMV-medaka Ara - and pCMV-medaka Arb - . COS-7 cells cultured in 24-multiwell plates (5.0 × 10 4 cells/well) were transfected with 400 ng/well of the PRE/ARE tk Luc reporter plasmid [78] , 0.8 ng/well of pRL-SV40 ( Renilla luciferase vector) as the internal control, and 80 ng/well of the expression vector for Ars, using 1.5 μL/well of TransFast transfection reagent (Promega, Tokyo, Japan). After 6 h of transfection, the cells were incubated for 12 h in Dulbecco’s modified Eagle’s medium with 10% charcoal-treated foetal bovine serum, either in the presence or absence of 10 −8 M 11KT (K-8250, Sigma-Aldrich, St. Louis, MO, USA). The reporter gene activities were determined using the dual-luciferase reporter assay system (Promega) with values normalised to pRL-induced activities (i.e. firefly luciferase activity/ Renilla luciferase activity). Each assay was performed in triplicates and repeated four times independently. The statistical significance of the reporter gene assay was analysed using two-sided Mann-Whitney U test by R version 4.2.0. Measurement of sex steroid levels Adult testes and whole brains of WT, ara KO, arb KO, and ar DKO males at ~6 months of age were collected 1 to 3 h after the onset of the light period, We judged that the 6 months old was proper to check the testicular function of medaka, because it has been shown that the plasma T and 11KT levels peak in male medaka at 8 months old [79] . 11KT, T, E1, and E2 were quantified in each testis or brain using liquid chromatography-tandem mass spectrometry (LC-MS/MS) at ASKA Pharma Medical Co. Ltd (Kanagawa, Japan) as described by Nishiike et al. [38] . Steroid levels are expressed as nanogrammes or picograms of each steroid per gram of wet tissue weight. Statistical differences between each mutant and the WT males were analysed using one-way ANOVA followed by two-sided Dunnett’s multiple comparison test in the ‘glht’ function of the R package multcomp version 1.4-20. Quantification of male fecundity Males (WT, ara KO, arb KO, and ar DKO) at six months of age were separated from females in the evening the day before the experiment. After measuring the body weight, the testes were removed, weighed, and homogenised with forceps for 1 min in 66 μL of ice-cold cryopreservation liquid (10% N,N-dimethylformamide) in foetal calf serum until the residual testis fragments became invisible. The obtained suspension was sucked into a glass capillary (Hirschmann disposable microcapillary, 10 μL/capillary, three capillaries for each testis) (Thermo Fisher Scientific, Waltham, MA, USA) and cryopreserved for artificial insemination according to the protocol provided by NBRP Medaka ( https://shigen.nig.ac.jp/medaka/medakabook/index.php ). Sperm suspension (4 μL) was mixed with 36 μL of ice-cold Iwamatsu’s balanced salt solution (BSS) by pipetting and immediately loaded into the sperm counting chamber (SC12-01-C, Leja Products B. V., Niew-Vennep, Netherlands). Sperm motility, average speed, and sperm concentration were examined using CASA (SMAS3 (ver.3.1.11.357), DITECT, Tokyo, Japan). For artificial insemination, 10 μL of sperm suspension in a glass capillary was thawed in 100 μL of ice-cold BSS and immediately added to the unfertilised eggs according to the protocol provided by NBRP Medaka. The GSI was calculated as follows: GSI (%) = gonad weight × 100/body weight. For the statistical analysis of the fertilisation rates, two-sided Dunnett’s multiple comparison in binomial GLMMs was conducted in R version 4.2.0 with the packages lme4 version 1.1-31 and multicomp version 1.4-20. The statistical significances of gonad/body weight, sperm motility test were analysed using one-way ANOVA followed by two-sided Dunnett’s multiple comparison test in the ‘glht' function of the R package multcomp version 1.4-20. Generation of Ar-FLAG-mClover3 knock-in (KI) medaka strains We generated KI medaka strains using a targeted gene trap approach mediated by the clustered regularly interspaced short palindromic repeats (CRISPR) and CRISPR-associated protein 9 (CRISPR/Cas9) system [80] . In this approach, the targeted insertion of a donor DNA vector harbouring a targeted genomic sequence can be induced by concurrent cleavage of the chromosomal target site and the circular donor DNA using the Cas9 ribonucleoprotein complex with a single guide RNA (gRNA) sequence. The donor vector for ara (pUC-Ara-3xFLAG-2A-mClover3 (a brighter and more photostable variant of green fluorescent protein) [81] includes a 484 bp segment of the partial genomic fragment consisting of a 322 bp segment of the 8th intron sequence and a 162 bp segment of the 9th exon sequence until just before the stop codon, while the vector for arb (pUC-Arb-3xFLAG-2A-mClover3) includes a 562 bp segment of the genomic fragment consisting of a 39 bp segment of the 7th exon sequence, 367 bp segment of the 7th intron sequence, and 156 bp segment of the 8th exon sequence. The partial genomic sequence of each vector was followed by in-frame insertion of a targeting cassette composed of a 3x FLAG sequence, P2A sequence derived from porcine teschovirus-1 [82] , the coding sequence of mClover3 from pNCS-mClover3 (Addgene Plasmid # 74236) [81] , and SV40 poly A signal (Fig. 6a ). Each donor vector was inserted into a gRNA-targeting site in the 8th or 7th intron of ara or arb , respectively. The resulting alleles could express mRNAs under the control of endogenous ar promoters, and the mRNAs are expected to be translated into two distinct proteins, namely, the C-terminal FLAG-tagged Ar and mClover3, owing to a ribosomal skipping by the P2A sequence [82] . Cas9 mRNA and gRNAs were generated as previously described [7] , [83] . Briefly, Cas9 mRNA was transcribed from the pCS2 + hSpCas9 vector using an mMessage mMachine SP6 Kit (Thermo Fisher Scientific). The sgRNAs were synthesised using the AmpliScribe T7-Flash Transcription Kit (Epicentre, Madison, WI, USA) with templates that were PCR-amplified using 57-mer oligonucleotides containing a T7 promoter sequence and a 20-mer sequence for a custom target (Supplementary Table 1 ). The donor plasmid vectors were extracted using an alkaline lysis miniprep approach, incubated at 55 °C for 30 min with 0.5% SDS and 0.8 µg/µL of proteinase K to eliminate the residual RNase activity, and then purified using NucleoSpin Gel and PCR Clean-up kit (MACHEREY-NAGEL) with the Buffer NTB. Microinjection of the OK-Cab strain into fertilised eggs was performed following a previously established method [84] . We injected ~1 nL of a mixture containing 100 ng/μL Cas9 mRNA, 10 ng/μL sgRNA, and 5 ng/μL donor plasmid. The targeted insertion of each donor vector in F 1 or later generations was examined by PCR genotyping using the primer pair GFP-127RV and ara-KI-5FW or arb-KI-5FW (Supplementary Table 1 ). Histological and immunohistochemical analyses Medaka tissues were fixed in 4% paraformaldehyde in PBS at 4 °C. The fixed tissues were decalcified using decalcifying solution B (041–22031, Fuji Film Wako, Osaka, Japan) for 48 h, dehydrated in graded methanol, embedded in paraffin, and cut into 6-μm-thick sections for Masson/trichrome staining and immunohistochemical analyses. Brain tissues were cut into 8-μm-thick sections and subjected to immunohistochemical analysis, as described previously [36] . Briefly, after antigen retrieval by incubating slides in 0.1 mM citrate buffer (pH 6.0) in an autoclave (121 °C) for 1 min, the sections were blocked for 1 h using 1xPBS containing 0.1% Tween 20, 2% BSA, and 2% foetal bovine serum, and incubated with anti-DDDDK-tag (FLAG) mouse mAb monoclonal antibody (M185-3L, MBL, Nagoya, Japan, 1:300 dilution) and anti-GFP D5.1XP rabbit mAb monoclonal antibody having cross-reactivity to the mClover3 (#2956, Cell Signaling, Danvers, MA, USA, 1:300 dilution) overnight at 4 °C. The sections were washed with 1xPBS with 0.1% Tween 20 (PBT), replaced with blocking buffer, and then incubated with Alexa 555-conjugated goat anti-mouse IgG(H + L), F(ab’) 2 fragment (#4409, Cell Signaling, 1:300 dilution), and Alexa 488-conjugated anti-rabbit IgG(H + L), F(ab’) 2 fragment (#4412, Cell Signaling, 1:300 dilution) for 1 h at room temperature. After counterstaining with the Cellstain DAPI solution (D523, Dojindo, Kumamoto, Japan), fluorescent signals were observed using an upright fluorescence microscope (Axioplan 2; Zeiss, Jena, Germany) or a confocal laser scanning microscope (FV1000, Olympus). GFP fluorescence in the whole body of adult fish was observed using a stereo fluorescent microscope FLUO III TM (Leica). Micrographs were taken using a digital charge-coupled device camera DP-73 (Olympus). Micro-computed tomography (micro-CT) and bone staining For micro-CT, the head parts were fixed as described above and then scanned using a Phoenix nanotom m (Baker Hughes, Houston, TX) at the JMC Corporation (Yokohama, Japan). For skeletal stains, Alcian blue/Alizarin red staining was performed as previously described [85] . The lengths of the fin and tooth of each fish were calculated using Adobe Photoshop CC 2019 (ver. 20.0.2) using a picture taken with a digital charge-coupled device camera (DP-73, Olympus) using a stereo microscope FLUO III TM (Leica). The statistical analyses of the tooth length and the number of papillary processes were conduceted one-way ANOVA followed by two-sided Dunnett’s multiple comparison test. The statistical significances in the fin lengths were analysed using two-sided Tukey’s multiple comparison test in the ‘glht’ function of the R package multcomp version 1.4-20. RNA isolation Each male was anaesthetised using 0.84% tricaine methanesulfonate (Sigma-Aldrich), and then the anal fins were separated into distal parts (distal three bone segments), anterior parts (the first to 10th fin rays counted from the anterior first fin ray), and posterior parts (the 11th fin ray to the posterior end where papillary processes generally develop on the fin rays). Total RNA was prepared from the posterior parts of the anal fin using an RNeasy Micro Kit (Qiagen, Hilden, Germany). WT, ara KO, and arb KO males were mated with a WT female and then anaesthetised immediately after courtship. ar DKO males were anaesthetised after 5 min of mating with a WT female. All matings were done within 1 h of the onset of the light period. The whole brain including the pituitary gland of each fish was collected from anaesthetised fish, and total RNA was purified using the RNeasy Plus Universal Kit (Qiagen). RNA-seq RNA-seq of the whole brain along with the pituitary gland was performed at Azenta (Tokyo, Japan). Briefly, cDNA libraries were prepared using MGIEasy RNA Directional Library Prep Set V2.0 (MGI Tech, Beijing, China) with 500 ng of total RNA after selection with the NEBNext Poly(A) mRNA Magnetic Isolation Module (New England Biolabs, Ipswich, MA, USA). The libraries were sequenced using the DNBSEQ-G400 platform (MGI Tech, Tokyo, Japan) with 2 × 150 bp paired-end reads. After adaptor and quality trimming using Trim Galore 0.6.4_dev with Cutadapt 1.18, transcripts were quantified with RNA-seq reads mapped to the transcriptome sequences of O. latipes (Hd-rR) (Ensembl 105; https://www.ensembl.org/ ) using salmon v1.3.0. The transcript counts were converted to gene-level counts using the R package tximport , and statistical analysis was performed using the R package edgeR v3.34.1. 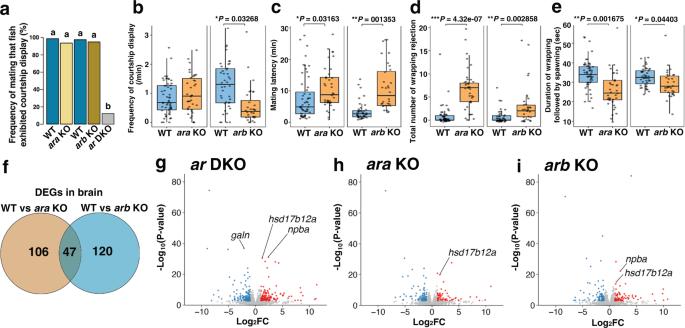Fig. 5: Botharaandarbare required for high male reproductive success. aPercentage of mating tests with different females in which a male exhibited courtship display within a 30 min test period. We used WT (n= 11, total 59 matings) andaraKO males (n= 14, total 76 matings) of the same litter, and WT (n= 6, total 40 matings) andarbKO males (n= 6, total 40 matings) of the same litter, andarDKO males (n= 10, total 43 matings) as mating partners for the WT females. The blue, light brown, dark brown, and grey colours indicate WT,araKO,arbKO, andarDKO, respectively. Means are shown. Different letters above the boxes indicate significantly different groups (P< 0.05, two-sidedfisher’s exact test with a Bonferroni correction).bFrequency of courtship displays before spawning.cTime required for spawning (mating latency).dTotal number of wrapping rejections by female.eDuration of wrapping followed by spawning. Forbtoe, we used WT (n= 11, total 55 mating) andaraKO males (n= 13, total 38 matings) of the same litter and WT (n= 6, total 42 matings) andarbKO males (n= 6, total 32 matings) of the same litter. The blue and brown colours in panelbtoeindicate WT andarKO males, respectively. Statistical differences were assessed by likelihood ratio test with two-sided alternative hypothesis in GLMMs (b–d) and LMMs (b–e) *P< 0.05, **P< 0.01, ***P< 0.001. In the box-plots, the centre line indicates the median, box limits indicate the upper and lower quartiles, the whiskers indicate 1.5× interquartile range, and the points are outliers. Source data and statistical data are provided as a Source Data file and Supplementary Table3, respectively.fRNA-seq of the whole brain with the pituitary in males. Venn diagram indicating overlap among inter-genotype differentially expressed genes (DEGs) (genes with >2-fold change in expression, false discovery rate (FDR) < 0.05).g–iVolcano plot with the log2fold-change on thex-axis and −log10of thepvalue on the y-axis in expression between WT andarDKO males (g), WT andaraKO males (h), and WT andarbKO males (i). Each dot represents a single gene with differently expressed genes (DEGs)coloured (FDR < 0.05). Thepvalues shown in the panels were calculated using two-sided Fisher’s exact test with no adjustments for the multiple comparisons. Of the 19,227 genes retained after filtering genes with lower expression with the ‘filterByExpr’ function, genes showing >2-fold change with <5% false discovery rate (FDR) in Fisher’s exact test were identified as differentially expressed genes between the WT and one of the Ar KO strains. GO enrichment analysis was conducted using ShinyGO 0.75 ( https://academic.oup.com/bioinformatics/article/36/8/2628/5688742 ) using the Ensembl gene IDs of the differentially expressed genes as input. Quantitative RT-PCR First-strand cDNA was transcribed from 500 ng of total RNA using SuperScript III (Thermo Scientific). The relative RNA equivalents for each sample were determined by normalising their levels to those of the internal control gene rpl7 [86] . Gene expression levels in the posterior part of anal fins of WT, ara KO, arb KO, and ar DKO males were quantified using 7500 real-time PCR with SYBR Green master mix (Thermo Scientific). The statistical significance of the differences was examined using one-way ANOVA followed by two-sided Dunnett’s multiple comparison test in the ‘glht’ function of the R package multcomp version 1.4-20. Primer sets used for the quantitative RT-PCR (qRT-PCR) analyses of lef1 and rpl7 were designed by Applied Biosystems Primer Express 2.0.0 (Thermo Fisher Scientific) and listed in Supplementary Table 1 . Behavioural assays To observe 1-to-1 mating behaviour, a male and a female were transferred into a single acrylic tank (200 mm length × 75 mm width × 150 mm height and filled with 2 L of water at 26.5 °C) and separated by a white plastic partition in the evening (18:00–19:00) of the day before the assay. After the onset of the light period (8:30–10:00), the behavioural trial was initiated by removing the partition. 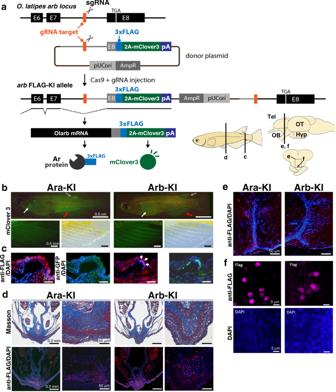Fig. 6: Visualisation of Ara and Arb expression in vivo by generating Ar-knock-in (KI) medaka strains. aStrategy for the generation of Ara and Arb KI medaka strains. We designed a gRNA targetingaraintron 8 andarbintron 7 (the last intron). In the donor plasmids, we cloned a genomic fragment beginning from the end of exon 8 ofaraand exon 7 ofarband ending just before the stop codon in the last exon, exon 9 ofara, and exon 8 (shown as black closed boxes with ‘E8’) ofarb, where the 3xFLAG sequences (shown as blue boxes) and a P2A (2A peptide from porcine teschovirus-1)-mClover3 cassette (shown as green boxes) was placed in the frame. Thus, endogenous Ara and Arb were expressed as FLAG fusion proteins. Both AR-FLAG and P2A-mClover3 were expected to be expressed under the control of the endogenous Ar promoter. To generate KI medaka, sgRNA (for genome digestion in the final intron), donor plasmid, and Cas9 mRNA were co-injected into one-cell-stage medaka embryos. After injection, concurrent cleavage of the targeted genomic locus and the donor plasmid resulted in the integration of donor plasmid DNA containing 3xFLAG-T2A-mClover3 by non-homologous end joining (NHEJ). The scheme shows the forward integration of 3xFLAG-T2A-mClover3.bExpression of mClover3 in adult males of the two knock-in medaka strains,araFLAG-2A-mClover3(Ara-KI) andarbFLAG-2A-mClover3(Arb-KI). White, grey, and red arrows indicate the regions adjacent to pectoral, dorsal, and anal fins, respectively (Ara-KI). White, grey, and red arrows indicate the pectoral, dorsal, and anal fins, respectively (Arb-KI).cImmunohistochemical detection of FLAG-tagged endogenous Ara and Arb in longitudinal sections of papillary processes of the anal fin (6 μm thickness). The merged images represent red fluorescence for immunostaining of FLAG (anti-DDDDK-tag mouse mAb monoclonal antibody), green fluorescence for immunostaining of mClover3 (anti-GFP D5.1XP rabbit mAb monoclonal antibody), and blue fluorescence for nuclear staining by DAPI. The medaka Arb-FLAG, but not Ara-FLAG, translocated into the nuclei of cells located in the distal tip of a bone nodule of papillary processes (marked by white arrows).dRepresentative micrographs of Masson/trichrome staining and immunohistochemical detection of FLAG-tagged endogenous Ara and Arb in adjacent sections of the urogenital region (8 μm thickness). Nuclear localisation of Ara-FLAG and Arb-FLAG was observed in the medulla ventral to the sperm duct, wherearDKO exhibited hyperplasia.e, fRepresentative micrographs showing immunohistochemical detection of FLAG-tagged endogenous Ara and Arb, and DAPI counterstaining in the brain (12 μm thickness).fshows a higher magnification of the POA. Nuclear localisation of both Ara-FLAG and Arb-FLAG was observed in the POA.n= 6 for Ara-KI and Arb-KI males, respectively. 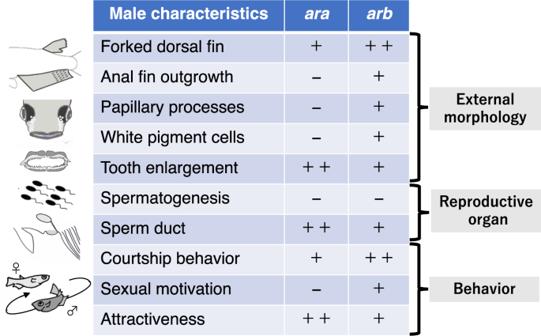Fig. 7: Summary of the contribution ofaraandarbto sexual characteristics. Based on the phenotypes ofaraKO andarbKO, the contribution of each of thearohnologs to male sexual characteristics is indicated by + or −. For the characteristics regulated by both, thearohnolog that predominantly controls them is indicated by ++. Mating behaviour was recorded until spawning using a digital video camera HDR-PJ800 (Sony, Tokyo, Japan). To exclude the effect of familiarity between the examined male and female, each test fish was crossed with another individual until the day prior to the assay. If the female lay eggs within 30 min of a behavioural trial, we analysed the number of courtship displays before spawning and the interval between the removal of the separator and successful egg spawning as mating latency, which is an indicator of female mate preference in medaka [7] . Wrapping behaviours that did not lead egg spawning were counted as wrapping rejections. If the wrapping led the spawning successfully, the period from the initiation of wrapping to the end of spawning was measured as a wrapping duration. We summarised the number of the mating tests for each analysis in Supplementary Table 2 . All videos in each dataset were analysed by a single viewer to ensure consistency. Statistical analysis for the frequency of reproduction and the frequency of mating that fish exhibited courtship display was conducted using two-sided fisher’s exact test with a Bonferroni correction in R version 4.2.0. For the other behavioural data, statistical analysis was conducted using GLMMs and LMMs in R version 4.2.0 with the package lme4 version 1.1.30. Poisson distributions with a log link function were used to analyse the number of courtship displays and wrapping rejections, whereas gamma distributions with a log link function were used for mating latency. The wrapping durations were analysed using LMMs. Genotypes and individual ID of males were included as fixed factors and random intercepts in each model. In the models for courtships, mating latency was included as a log-linear offset to standardise the number of events per unit time. The significant effect of the male genotype in each model was evaluated using the likelihood ratio test between the full and null models, excluding the fixed factor. To directly measure the female mate preference to WT male or ar KO male, we performed round-robin tournaments using five WT males and five ar KO males, that is, a total of 25 combinations of mate choice test for each ar KO strain. The scores were given as the frequency with which each male mated with a female. Similar to the 1-to-1 mating behavioural analysis above, this mate choice test was initiated after the onset of the light period (8:30–10:00). A WT male and an ara KO or arb KO male were transferred to a single tank with a WT female. Then, their behavioural interactions were recorded until spawning. Each male individual was distinguished by the pigment pattern of the melanophores and fin shape. A male individual that led to egg spawning was judged as a successful mating partner under observation of each video recording. If the female did not lay eggs within 1 h of a behavioural trial, we judged the trial to be a draw. Effects of each ar mutation on the mate behaviour were statistically analysed using the chi-squared ( χ 2 ) test of independence in R version 4.2.0 with the package lme4 version 1.1.30. To measure the female fecundity of the ar KO strains, a female of WT, ara KO, arb KO, or ar DKO strains was transferred into a test tank with a WT male, and they were separated by a partition on the day before the test, as described above. After removing the separator in the morning of the test day, we analysed whether the females spawned the eggs. If the female successfully spawned, the total number of eggs obtained and their fertilisation rates were quantified. This test was repeated for 10 consecutive days by exchanging the males daily. Reporting summary Further information on research design is available in the Nature Portfolio Reporting Summary linked to this article.